Trinucleotide duplex formation inside a confined nanospace under supercooled conditions Self-assembly of nucleotides of fewer than three base pairs is often found in protein–nucleotide conjugations, despite their energetic instability, and is regarded as the potential starting point for the creation of artificial hydrogen-bonded supramolecular complexes. Here we report duplex formation of 3-mer DNA fragments confined within silica mesopores modified with a positively charged trimethyl aminopropyl monolayer, and their further stabilization under supercooled conditions ( T <273 K). We load 3-mer DNA fragments with donor- or acceptor-dye into modified silica mesopores and examine their hybridization behaviours using FRET measurements. The FRET results clearly reveal that efficient duplex formation through at least two A-T base pairs can be achieved at 233 K. Enthalpy changes for duplex formation are found to be nearly equal between complementary and single-mismatched 3-mer DNA duplexes. These results confirm confined mesoscale cavities to be a novel low-temperature reaction space for hydrogen-bonded supramolecular complexes. Self-organization of short nucleotides is energetically disfavoured in dilute aqueous solutions [1] , [2] ; accomplishing this process in an artificial system remains a challenging task that draws on molecular biology, supramolecular chemistry and nanoscience. One recently successful approach has involved the use of hydrophobic cavities in pyrazine-pillared coordination cages dispersed in water [3] . Hydrogen-bonded base pairing in a hydrophobic cavity isolated from the water phase has been proposed to be responsible for the stabilization of anti-Hoogsteen-type base pairs of minimal (mono- and di-) nucleotides. The use of molecular crowding [4] , [5] or binding ligands [6] , [7] are also fruitful strategies for assisting self-organization. These approaches rely on the structural and/or thermodynamic stabilization of hydrogen-bonded base pairing in specific environments that mimic nucleotide–protein conjugates in the living cell [8] . The design of artificial reaction spaces to achieve significant stability gains has therefore been a major focus of research into the self-organization of short nucleotides. Up to now, however, no artificial system has been developed that promotes the effective formation of trinucleotide duplexes. Mesoporous silica synthesized by supramolecular templating approach has uniform cylindrical pores of approximately the diameter of oligonucleotide duplexes (~2 nm; refs 9 , 10 , 11 , 12 ). Functional groups attached to the inner surfaces of these pores can be used to fine-tune surface character, effective pore diameter and the microenvironment inside the pore [13] . Mesoporous silica pores thus provide a potentially useful confined nanospace for stabilizing short nucleotide duplexes. We also employ supercooled confined water [14] , [15] , [16] , [17] as part of our strategy to achieve efficient duplex formation. The melting temperatures ( T m ) of short DNA duplexes is far <273 K; for example, the T m values for oligo d[A:T] n DNA parallel-stranded DNA duplexes ( n =number of bases) predicted using the nearest-neighbour model [18] are 257 K ( n =4) and 222 K ( n =3). These T m values imply that duplex formation of short DNA fragments can be accelerated in supercooled water ( T <273 K), if the solvent water can be deeply and reliably supercooled [19] . It is difficult to control supercooled water in bulk systems; however, water confined inside mesoporous silica can be deeply supercooled and maintains its fluidity at temperatures above 223 K (refs 14 , 15 , 16 , 17 ). Silica mesopores, therefore, can be regarded as a novel low-temperature reaction space for accelerating duplex formation of short DNA fragments. In the present study, we examined duplex formation of 3-mer DNA fragments inside a silica mesopore modified with a trimethyl aminopropyl (TMAP) monolayer over the temperature range of 233–303 K by means of FRET measurements. The results confirm that efficient hybridization of 3-mer DNA duplexes through at least two A-T base pairs can be accomplished inside the TMAP-modified silica mesopore under supercooled conditions ( T <273 K). Characterization of TMAP-HMM and DNA location A hybrid mesoporous membrane (HMM) composed of mesoporous silica and porous anodic alumina membrane was prepared using the aspiration method [20] , [21] . A dense TMAP monolayer (1.4 molecules nm −2 ) was formed on the inner pore surface of the mesoporous silica using the post-grafting method ( Fig. 1 ) [22] . The resulting TMAP-modified HMM (TMAP-HMM) has a silica mesophase with a quasi-hexagonal pore arrangement ( Supplementary Fig. 1 ). The effective diameter of the TMAP-modified silica pore is 2.4 nm. 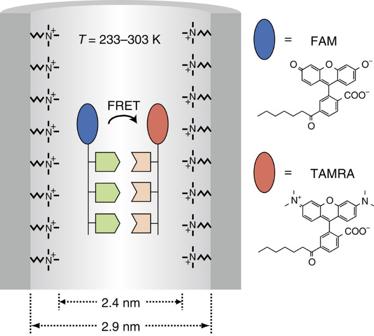Figure 1: Schematic illustration of 3-bp DNA duplex inside a pore. The end of the 3-mer DNA fragment is modified with FAM (5′ end) or TAMRA (3′ end) for FRET observation. The hybridization equilibria of 3-mer DNA fragments confined inside a TMAP-modified silica mesopore are examined over temperature range of 233–303 K. The structural parameters of HMM and TMAP-HMM are summarized in Table 1 . Figure 1: Schematic illustration of 3-bp DNA duplex inside a pore. The end of the 3-mer DNA fragment is modified with FAM (5′ end) or TAMRA (3′ end) for FRET observation. The hybridization equilibria of 3-mer DNA fragments confined inside a TMAP-modified silica mesopore are examined over temperature range of 233–303 K. Full size image Table 1 Structural parameters for HMM and TMAP-HMM. Full size table The 5′ FAM-modified DNA and 3′ TAMRA-modified DNA fragments, together with water molecules, were introduced into the TMAP-modified silica pores at room temperature; their hybridization behaviour was then examined using FRET measurements. 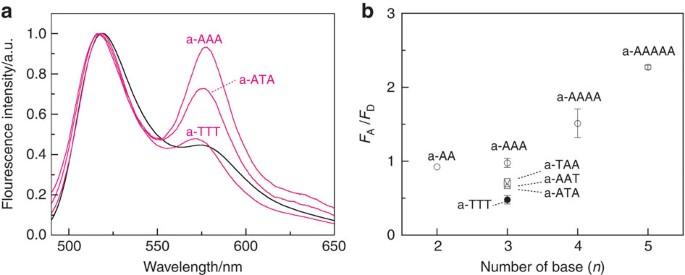Figure 2: FRET responses for TMAP-HMM containing DNA fragments at 273 K. (a) Typical fluorescence spectra for TMAP-HMM (magenta lines) containing d-TTT and a-NNN (NNN=AAA, ATA or TTT). The fluorescence intensities were normalized to the peak intensities of the donor band. The black line represents spectrum for d-TTT and a-AAA in bulk water at 273 K. (b) Fluorescence intensity ratio of acceptor to donor bands (FA/FD) observed for TMAP-HMMs containingn-mer DNA pairs (d-Tn/a-An) and mismatched 3-mer DNA pairs (d-TTT/a-TAA, a-AAT, a-ATA and a-TTT). The standard deviations (error bars) for each experimental data are obtained from at least three independent measurements. The abbreviation of sample DNAs, sequences and the amounts of DNA inside the pores are summarized in Table 2 . The amounts of DNA adsorbed at the TMAP-HMM were about seven times greater than those found for a porous anodic alumina membrane modified with TMAP groups. This result confirms that the DNA fragments are predominantly located inside the TMAP-modified silica pores. Table 2 Amounts of M DNA and V DNA inside the TMAP-modified silica pores. Full size table FRET responses of DNA fragments inside the pores Figure 2a shows normalized fluorescence spectra of TMAP-HMMs containing both d-TTT and a-NNN (NNN=AAA, ATA or TTT) inside the pores at 273 K, together with that for bulk water containing d-TTT and a-AAA. For the bulk water system, acceptor emission was too weak because d-TTT and a-AAA generally do not form a duplex in bulk water. On the other hand, significant acceptor emission was observed when a complementary DNA pair (d-TTT and a-AAA) was confined inside the pores. In the time-resolved fluorescence measurements, the confined DNA pair exhibited quenching of the donor emission accompanied by a rise, after a delay, of the acceptor emission ( Supplementary Fig. 2 ). These results suggest that hybridization of d-TTT and a-AAA produced FRET inside the pores. This view is supported by the fact of sequence and base number dependencies of fluorescence intensity ratio of acceptor to donor bands ( F A / F D ). The F A / F D value for complementary 3-mer DNA pair was stronger than those for a single-mismatched 3-mer DNA pair ( Fig. 2b ). In addition, a stronger F A / F D value was observed for longer DNA pairs. These sequences and base number dependencies of F A / F D mean that the hybridization efficiency rises on increasing the number of A-T base pairs to form a duplex, which agrees with the well-known stability of DNA duplexes through A-T Watson–Crick hydrogen-bonding [1] , [18] . It can thus be concluded that the FRET response is ascribed to the hybridization of a 3-mer DNA duplex. Figure 2: FRET responses for TMAP-HMM containing DNA fragments at 273 K. ( a ) Typical fluorescence spectra for TMAP-HMM (magenta lines) containing d-TTT and a-NNN (NNN=AAA, ATA or TTT). The fluorescence intensities were normalized to the peak intensities of the donor band. The black line represents spectrum for d-TTT and a-AAA in bulk water at 273 K. ( b ) Fluorescence intensity ratio of acceptor to donor bands ( F A / F D ) observed for TMAP-HMMs containing n -mer DNA pairs (d-T n /a-A n ) and mismatched 3-mer DNA pairs (d-TTT/a-TAA, a-AAT, a-ATA and a-TTT). The standard deviations (error bars) for each experimental data are obtained from at least three independent measurements. 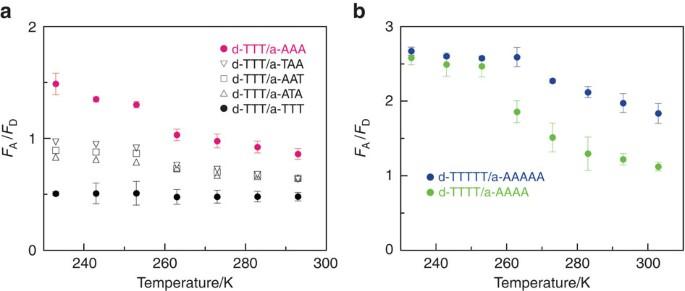Figure 3: FRET responses at temperature between 293 and 233 K. (a) Temperature dependencies ofFA/FDfor 3-mer DNA pairs confined inside the pores. (b) Temperature dependencies ofFA/FDfor 4- and 5-mer DNA pairs confined inside the pores. The s.d. (error bars) for each experimental data are obtained from at least three independent measurements. Full size image The effect of temperature on the hybridization of 3-mer DNA fragments was examined over the temperature range of 233–303 K. Figure 3a summarizes the temperature dependencies of F A / F D for 3-mer DNA pairs in bulk water and inside pores. When a non-complementary 3-mer DNA pair (d-TTT and a-TTT) was confined inside the pore, no significant change in F A / F D with temperature was observed, and the average value of F A / F D was 0.49±0.20, close to that found for the non-complementary 3-mer DNA pair in bulk water (0.45). This result indicates that, due to the lack of an A-T base pair, no hybridization of non-complementary 3-mer DNA fragments took place inside the pores. On the other hand, complementary (d-TTT and a-AAA) and single-mismatched (d-TTT/a-NNN: NNN=TAA, ATA, AAT) 3-mer DNA pairs inside the pore exhibited a clear increase in F A / F D with decreasing temperature. These temperature dependencies of F A / F D are ascribed to the acceleration of the duplex formation under the supercooled conditions (233–273 K) because the hybridization is an exothermic reaction [18] . Since the change in F A / F D with temperature is reversible without hysteresis ( Supplementary Fig. 3 ), it appears that a hybridization equilibrium of 3-mer DNA fragments is established inside the pores. It has been reported that water confined inside aminopropyl-modified silica mesopores (effective pore diameter=2.3 nm) does not freeze, and its microviscosity remains <12 mPa s at temperatures >223 K (ref. 17 ). Similarly, water confined inside a TMAP-modified silica mesopore can be regarded as a liquid above 233 K. The presence of fluidic water under supercooled conditions would allow the diffusion of DNA fragments to hybridize/dehybridize, resulting in the establishment of a hybridization equilibrium. Figure 3: FRET responses at temperature between 293 and 233 K. ( a ) Temperature dependencies of F A / F D for 3-mer DNA pairs confined inside the pores. ( b ) Temperature dependencies of F A / F D for 4- and 5-mer DNA pairs confined inside the pores. The s.d. (error bars) for each experimental data are obtained from at least three independent measurements. Full size image Figure 3b shows the temperature dependency of F A / F D on complementary 4- and 5-mer DNA pairs inside pores. For the 3-mer DNA pair, F A / F D gradually increases with falling temperature over the observed temperature range ( Fig. 3a ). For 4- and 5-mer DNA fragments, on the other hand, the temperature dependency of F A / F D takes the form of a sigmoidal curve, resembling the often-observed DNA melting curve in bulk water. The F A / F D value before the inflection temperature tends to be larger for longer DNA fragments. The F A / F D value in the quasi-plateau region is almost the same regardless of the number of bases. These features for 4- and 5-mer DNA pairs suggest that the hybridization equilibria are completed below the inflection temperature. For 3-mer DNA fragments, therefore, we conclude that the hybridization equilibrium is not completed within the observed temperature range. Estimation of assembled fraction F A / F D values were used for an estimation of assembled fraction ( θ ) of the FAM- and TAMRA-modified DNA fragments on the basis of a simple two-state model [23] , which is constructed assuming that only the DNA duplex exhibits a FRET response. In the two-state model, the relationship between F A / F D and θ is described by equation (1) where a and b are minimal and maximal F A / F D values, respectively. The minimal and maximal F A / F D values correspond to completely dissociated and hybridized structures of DNA fragments, respectively. The d term is the ratio of F A values for dissociated and hybridized structures. The details in the derivation of equation (1) are described in the Supplementary Note 1 . In a bulk water system, d-T 10 /a-A 10 pair exhibited clear FRET response ( Fig. 4a ), and analysis of the FRET response on the basis of a conventional donor-quenching approach [23] ( Supplementary Note 2 ) confirmed that θ of d-T 10 /a-A 10 pair was almost 1 below 278 K ( Fig. 4b ). This efficient hybridization was supported by isothermal calorimetry studies ( Supplementary Fig. 4 ). The θ values shown in Fig. 4b agree closely with those estimated from the analysis of F A / F D values using equation (1); the correlation coefficient is 0.994 ( Supplementary Fig. 5 ). Accordingly, equation (1) can be used to make an estimate of the assembled fraction. In general, the FRET response depends on various factors, including donor–acceptor distance, spectral overlap of donor emission and acceptor absorption, dipole orientation factor and the microenvironments around the donor and acceptor dyes [24] , [25] ; however, experimental determination of these factors inside the pore is problematic. In the 3-mer DNA pairs inside pores, therefore, the assembled fraction was approximately estimated using the b and d terms obtained in the bulk system ( Fig. 4a ). The value of a was derived from the average F A / F D value for non-complementary (d-TTT/a-TTT) DNA pairs inside the pores. The a , b and d values are 0.49, 3.2 and 0.069, respectively. 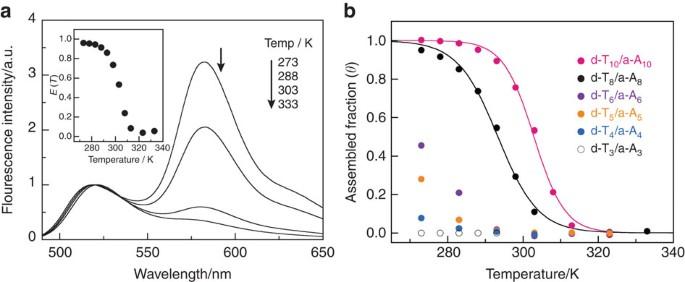Figure 4: Duplex formation of d-Tn/a-Anin bulk water. (a) Typical fluorescence spectra of d-T10/a-A10pair in bulk water ([DNA], 10 μM; [NaCl], 100 mM; [sodium cacodylate buffer], 10 mM; [EDTA], 1 mM, at pH 7.0). The fluorescence intensities were normalized to the peak intensities of the donor band. Inset of (a) shows FRET efficiencies of d-T10/a-A10pair. (b) Assembled fractions ofn-mer DNA pairs (d-Tn/a-An) estimated by donor-quenching approach. Figure 4: Duplex formation of d-T n /a-A n in bulk water. ( a ) Typical fluorescence spectra of d-T 10 /a-A 10 pair in bulk water ([DNA], 10 μM; [NaCl], 100 mM; [sodium cacodylate buffer], 10 mM; [EDTA], 1 mM, at pH 7.0). The fluorescence intensities were normalized to the peak intensities of the donor band. Inset of ( a ) shows FRET efficiencies of d-T 10 /a-A 10 pair. ( b ) Assembled fractions of n -mer DNA pairs (d-T n /a-A n ) estimated by donor-quenching approach. Full size image The assembled fractions for confined systems and bulk water systems are shown in Figs 4b and 5a , respectively. At the lowest temperature for bulk water systems (273 K), the assembled fraction is smaller for shorter DNA pairs (d-T n /a-A n ; n =number of bases). Hybridization of 3-mer DNA pairs is rare in the bulk water system. In the confined system, on the other hand, complementary 3-mer DNA pairs (d-TTT/a-AAA) form duplexes at temperatures even higher than 273 K, and their assembled fraction rises to ~0.9 on decreasing the temperature to 233 K. Even for single-mismatched DNA pairs, assembled fractions were ~0.7 at 233 K. Efficient duplex formation of 3-mer DNA pairs can thus be accomplished inside TMAP-modified silica mesopores under supercooled conditions. 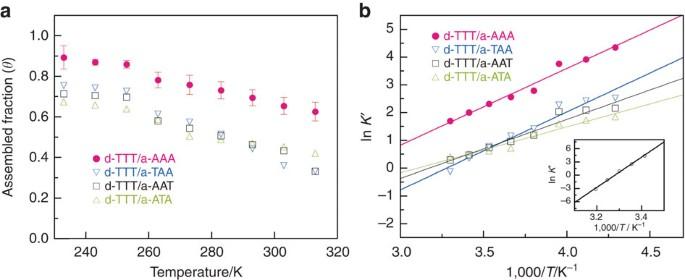Figure 5: Duplex formations of 3-mer DNA pairs for confined systems. (a) Assembled fractions of 3-mer DNA pairs inside TMAP-modified silica mesopores. The assembled fractions for TMAP-HMM systems were estimated using equation (1). (b) van’t Hoff plots for the hybridization of 3-mer DNA pairs inside the pore. Inset ofbshows a van’t Hoff plot of d-T10/a-A10pair in bulk water. The solid lines are results by best fit using equation (2). Figure 5: Duplex formations of 3-mer DNA pairs for confined systems. ( a ) Assembled fractions of 3-mer DNA pairs inside TMAP-modified silica mesopores. The assembled fractions for TMAP-HMM systems were estimated using equation (1). ( b ) van’t Hoff plots for the hybridization of 3-mer DNA pairs inside the pore. Inset of b shows a van’t Hoff plot of d-T 10 /a-A 10 pair in bulk water. The solid lines are results by best fit using equation (2). Full size image Duplex formation of 3-mer DNA fragments For the confined system, the hybridization equilibrium of 4-mer DNA pair (d-TTTT/a-AAAA) is completed at 233 K as shown in Fig. 3b , suggesting that the assembled fraction of the 4-mer DNA pair at 233 K can be assumed to be 1. On the basis of this assumption, from the fluorescence spectra of d-TTTT/a-AAAA pair and d-TTTT inside the pores at 233 K ( Supplementary Fig. 6 ), the FRET efficiency and the donor–acceptor distance for the duplex of 4-mer DNA pair were estimated to be 0.95 and 2.8 nm (Förester distance=4.5 nm (ref. 24 )), respectively ( Supplementary Note 3 ). These values are consistent with those for duplex of 10-mer DNA pair (d-T 10 /a-A 10 ) in bulk water (0.96 and 2.6 nm, inset of Fig. 4a ). These results suggest that donor–acceptor configuration in the duplex formed inside the pore is the same as that for the 10-mer DNA duplex. Since the FRET efficiencies for parallel and antiparallel duplexes of d-T 10 /a-A 10 are respectively expected to be ~0.2 and >0.9 (ref. 24 ), the FRET efficiency of 0.96 indicates the formation of antiparallel duplex of d-T 10 /a-A 10 in bulk water. In the theoretical study of d(A:T) n DNA duplexes ( n =5 to 15; ref. 26 ), it was reported that the parallel duplex was less stable than the antiparallel duplex. It can therefore be considered that the short DNA fragments (3-mer and 4-mer DNA fragments) also form a stable antiparallel duplex inside the pore. The formation of the stable antiparallel duplex inside the pore brings the donor and acceptor in close proximity, yielding high FRET efficiency (0.95). This view is supported by the fact of efficient hybridization of d-TTG/a-AAC pair and d-TGT/a-ACA pair inside the pores. d-TTG and d-TGT are 5′ FAM-modified DNA fragments, and a-AAC and a-ACA are 3′ TAMRA-modified DNA fragments. The TMAP-HMM containing d-TTG/a-AAC pair or d-TGT/a-ACA pair exhibited clear acceptor emission at 273 K ( Supplementary Figs 7 and 8 ), and analysis of the F A / F D values provided similar assembled fractions for both DNA pairs; 0.83 for d-TTG/a-AAC pair and 0.82 for d-TGT/a-ACA pair ( Supplementary Note 4 ). The assembled fractions for d-TGT/a-ACA pair and d-TTG/a-AAC pair were larger than that for d-TTT/a-AAA pair (0.76), as predicted by the nearest-neighbour model for antiparallel DNA duplexes [18] . If parallel duplex is predominantly formed inside the pore, the hybridization efficiency for the d-TTG/a-AAC pair should be much lower than that for the d-TGT/a-ACA pair because only one non-Watson–Crick base pair is responsible for the parallel duplex formation of d-TTG/a-AAC. It therefore can be concluded that the 3-mer DNA pairs form an antiparallel duplex inside the pore. Likely reasons for this efficient duplex formation are related to the presence of a dense TMAP layer at the inner pore surface. The apparent ionic strength inside the pore was estimated to be 3.5 M by assuming that the quaternary amine groups and their counter anions contribute to the ionic strength. The polarity inside the pore is lower than that for bulk water [27] . These environments inside the pore are favoured for base pairing of DNA [4] , [5] . Spatial confinement inside a small cylindrical cavity (effective diameter=2.4 nm) surrounded by a positively charged TMAP layer also appears to contribute to the stabilization of DNA duplexes (see Fig. 1 ) [7] . The concentration of the 3-mer DNA pair inside the pore is another major reason for the high assembled fraction inside the pore. As shown in Table 2 , the average volume occupied by a single 3-mer DNA is ~1.0 × 10 3 nm 3 molecule −1 , two orders of magnitude smaller than that in 10 μM DNA bulk solution (1.7 × 10 5 nm 3 molecule −1 ). We believe that the combination of these specific environments, the spatial confinement effect and the high DNA concentration, results in the formation of 3-mer DNA duplexes inside the pore. Further stabilization under supercooled conditions improve the hybridization efficiencies of 3-mer DNA duplexes inside the pore, because the water confined within mesoporous silica can be deeply supercooled [14] , [15] , [16] , [17] . The assembled fractions of single-mismatched 3-mer DNA pairs appear to be independent of mismatch position ( Fig. 5a ), implying that the position of the mismatch does not influence the stability of the mismatched DNA duplex. The differences in assembled fraction between complementary and single-mismatched 3-mer DNA pairs are not very great: the assembled fractions for single-mismatched 3-mer DNA pairs are only ~1.4 times smaller than those for complementary ones at 273 K. On the basis of the FRET response of 2-mer DNA pairs (d-TT/a-AA) inside the pore ( Fig. 2b ), the assembled fraction for 2-mer DNA pairs inside the pore was estimated to be 0.73 at 273 K. These results confirm that efficient hybridization of 3-mer DNA duplexes through at least two A-T base pairs can be accomplished within a TMAP-modified silica mesopore. Enthalpy changes for duplex formation of 3-mer DNA fragments In the simple DNA–DNA hybridization model, the enthalpy (Δ H ) and entropy (Δ S ) changes for the duplex formation can be estimated from θ values [23] : where C 0 is the total concentration of DNA fragments in the system. Since the linear relationship between K ' and 1/ T could be identified as 3-mer DNA pairs inside the pores ( Fig. 5b ), the enthalpy changes were estimated by fitting data to equation (2). In the present study, the amounts of DNA molecules confined inside the pores were estimated. However, these amounts were not directly used to calculate the concentration of DNA within the pores because the definition of the effective volume for the duplex formation is difficult. We therefore did not estimate the entropy changes. As listed in Table 3 , the enthalpy changes for 3-mer DNA pairs confined inside the pore are one order of magnitude smaller than those for 10-mer DNA pairs (d-T 10 /a-A 10 ) in bulk water. The small enthalpy changes for 3-mer DNA pairs may be qualitatively explained by the smaller number of A-T base pairs and the lack of cooperative interactions [2] , [18] . In the nearest-neighbour model [18] , the change in Δ H for a d-T n /a-A n pair is −8 kcal mol −1 per single base pair. The energy of the H-bonds in one A-T base pair was estimated to be ~−12 kcal mol −1 using ab initio molecular orbital simulation [28] . In the light of these energy values, the difference in Δ H values between complementary and single-mismatched 3-mer DNA pairs appears to be small, with the maximum difference in Δ H being 2.3 kcal mol −1 ( Table 3 ). This small difference in Δ H is likely responsible for the relatively efficient hybridization of single-mismatched 3-mer DNA pairs inside the pore. Table 3 Enthalpy changes for the hybridization of DNA fragments. Full size table In DNA duplexes with T·T mismatch, mismatched thymine bases tend to be intercalated in the duplex and to form a wobble base pair involving two imino to carbonyl hydrogen bonds [29] . In bulk water system, however, the wobble base pair is not stable and its structure is fluctuated particularly at high temperature [29] , [30] . In the present confined system, 3-bp DNA duplex is tightly confined inside the cylindrical pore with 2.4 nm of effective pore diameter. Since fluctuation of the mismatched thymine is restricted due to the spatial confinement, it can be considered that the mismatched thymine bases are forced to stay in the duplex. The hydrogen bonds between mismatched thymine bases and stacking between mismatched thymine and neighbouring bases might effectively stabilize the single-mismatched duplex confined inside the pore. Self-assembly of nucleotides with a few base pairs has an important roll in biological systems. For example, codon–anticodon duplex within ribosome is 2–3 base pair stretch of A-form helix [31] . In duplex formation of oligonucleotide, double helix zips up after formation of a nucleus composed of 2–3 hydrogen-bonded base pairs [32] , [33] . The present study confirmed that hybridization of short nucleotides could be controlled inside the TMAP-modified silica mesopore. The meso-scale cavity including the present silica pore can serve as novel reaction space for structural study as well as dynamic study of short nucleotide assembly. In conclusion, we have demonstrated for the first time that duplexes of 3-mer DNA fragments can be formed with high efficiency inside a TMAP-modified silica mesopore, and that the hybridization equilibrium can be improved under supercooled conditions (233–273 K). The results obtained in this study suggest new strategies for designing hydrogen-bonded supramolecular networks within confined nanospaces. The stabilities of 3-bp DNA duplexes with/without single-base mismatching will also contribute to comprehensive understanding of the self-assembly process of nucleotides in protein–nucleotide conjugations. Preparation and characterization of TMAP-HMM The details of TMAP-HMM preparation are described in our previous papers [20] , [21] , [22] . A mixture of ethanol (7.68 g), TEOS (11.57 g) and 1 ml of HCl aqueous solution (2.8 mM) was refluxed at 60 °C for 90 min. Then, ethanol (15 g), 4 ml of HCl solution (55 mM) and cetyltrimethylammonium bromide (1.52 g) were added to the refluxed solution, which was stirred for 30 min to give the precursor solution. Porous anodic alumina membranes (pore diameter=~200 nm, thickness=~60 μm, diameter of membrane=25 or 47 mm) were obtained from Whatman (Anodisc). The precursor solution was introduced into the columnar alumina pores under moderate aspiration [20] , [21] . After calcination to remove the template surfactant, the calcined membrane (HMM) was immersed in a mixture of 8.9 ml of 1,4-dioxane, 20.8 ml of 1-hexanol, and 0.3 ml of N -trimethoxysilylpropyl- N,N,N -trimethylammonium chloride (50 wt% in methanol) and heated under reflux for 12 h at 102 °C (ref. 22 ). After refluxing, the TMAP-modified HMM was rinsed with acetone and water three times each. The resulting TMAP-HMM was characterized by nitrogen adsorption isotherms and X-ray diffraction (XRD) measurements. Nitrogen adsorption and desorption isotherms were measured on a Micrometrics ASAP 2020 instrument. The specific surface area was calculated using the multiple-point Brunauer–Emmett–Teller (BET) method, and the pore distribution was calculated from the adsorption branch of the isotherm using the Barrett–Joyner–Halenda (BJH) method. The XRD patterns of the HMM and TMAP-HMM were recorded on a MAC Science/Bruker M21X with CuK α radiation. The diffraction pattern was recorded in the 2 θ range of 0.51°–10°, with a 2 θ step size of 0.01°, running at a voltage of 45 kV. The HMM and TMAP-HMM were ground in an agate mortar before the elemental analysis and XRD measurements. Yanaco model CHN MT-6 elemental analyzer was used to determine the nitrogen weight percentages in the TMAP-HMM. Introduction of DNA fragments within TMAP-HMM 5′ FAM-modified DNA and 3′ TAMRA-modified DNA fragments ( Fig. 1 ) were custom-synthesized and HPLC-purified (>97%) by Nihon Gene Research Laboratories Inc. The DNA fragments were introduced into the TMAP-modified silica mesopores within TMAP-HMM by exposure to a droplet of DNA solution for 6 h under saturated water vapour conditions. The DNA solution was buffered to pH 7.0 with 10 mM sodium cacodylate containing 100 mM NaCl and 1.0 mM EDTA and 10 μM each of 5′ FAM-modified DNA and 3′ TAMRA-modified DNA fragments. After introduction of DNA to the pores, the droplet of DNA solution was collected and subjected to absorption spectrum measurement to estimate the amount of DNA introduced. The abbreviations for sample DNAs, sequences and the amounts of DNA inside the pores are summarized in Table 2 . The TMAP-HMM with DNA fragments was rinsed with buffer solution (10 mM sodium cacodylate containing 100 mM NaCl and 1.0 mM EDTA, pH 7.0) to remove any DNA adsorbed to the outer membrane surface. Fluorescence measurements The TMAP-HMM with DNA fragments was fixed on a Teflon holder in a quartz cell (1 cm × 1 cm) filled with heptane to prevent evaporation of water inside the silica mesopores during the fluorescence measurements [17] , [19] . The steady-state fluorescence spectra were measured using a spectrofluorophotometer (FP-6500, JASCO) equipped with a cryostat (CoolSpek USP-203, Unisoku). The excitation wavelength was 455 nm for all fluorescence measurements. The standard deviations (error bars) for each experimental data were obtained from at least three independent measurements. The time-resolved fluorescence measurement system was composed of mode-locked titanium:sapphire laser (Spectra-Physics, Mai Tai; ~100 fs, 80 MHz) and streak scope (Hamamatsu, C10627). The second harmonic (450 nm) of the fundamental laser beam was used as an excitation source. The excitation laser beam was shone on a TMA-HMM containing DNA fragment in a quartz cell and fluorecence from it was introduced to the streak scope. The instrumental time resolution of the present system was ~100 ps at 10 ns full scale. Fluorescence decay profiles for donor band (510–530 nm) and acceptor band (565–595 nm) were observed for TMAP-HMMs containing d-TTT only, a-AAA only and complementary DNA pair (d-TTT/a-AAA), respectively. The time-resolved fluorescence experiments were performed at a room temperature (298 K). How to cite this article: Arafune, H. et al. Trinucleotide duplex formation inside a confined nanospace under supercooled conditions. Nat. Commun. 6:5151 doi: 10.1038/ncomms6151 (2014).